The role of chalcogen vacancies for atomic defect emission in MoS2 For two-dimensional (2D) layered semiconductors, control over atomic defects and understanding of their electronic and optical functionality represent major challenges towards developing a mature semiconductor technology using such materials. Here, we correlate generation, optical spectroscopy, atomic resolution imaging, and ab initio theory of chalcogen vacancies in monolayer MoS 2 . Chalcogen vacancies are selectively generated by in-vacuo annealing, but also focused ion beam exposure. The defect generation rate, atomic imaging and the optical signatures support this claim. We discriminate the narrow linewidth photoluminescence signatures of vacancies, resulting predominantly from localized defect orbitals, from broad luminescence features in the same spectral range, resulting from adsorbates. Vacancies can be patterned with a precision below 10 nm by ion beams, show single photon emission, and open the possibility for advanced defect engineering of 2D semiconductors at the ultimate scale. Control over atomic defects is the foundation of today’s semiconductor technology. For two-dimensional van der Waals semiconductors, the term “defect engineering” has been coined to suggest that, by introducing defects, these materials can be engineered beyond the established concepts of doping or alloying [1] , enabling advanced functionality, such as single photon sources [2] , [3] or photocatalysis with chemical specificity [1] . Nevertheless, the microscopic understanding of defect-related modifications remains elusive due to a lack of thorough correlation between atomic structure and resulting macroscopic electronic and optical properties. Combing controlled defect engineering with optical spectroscopy as well as atomic imaging and ab initio theory, we identify the optical signature of pristine chalcogen vacancies in MoS 2 . Vacancies introduce a deep center with sharp optical emission, markedly different from previously observed broad luminescence bands [4] , [5] , [6] , [7] , [8] . Comparing annealed vs . He-ion treated MoS 2 , we establish that the recently discovered single-photon emitters in He-ion irradiated MoS 2 originate from chalcogen vacancies [3] . The latter can be deterministically created with a precision below 10 nm [9] , underscoring the potential of defect engineering for two-dimensional (quantum-) optoelectronics. In semiconductors, the interaction of free excitons with the Coulomb potential of lattice defects results in localized defect-exciton complexes [10] . In the traditional picture, exciton localization at shallow defects introduces an additional binding energy. Therefore, optical signatures of defects lie energetically below the free exciton [10] . Defect levels deep inside the band gap provide further relaxation pathways at even lower transition energies [10] . Since in two-dimensional (2D) semiconducting transition metal dichalcogenides, including MoS 2 , MoSe 2 , WS 2 , and WSe 2 , the screening of the defect potential is weak, and also the exciton Bohr radius is small (~ 2–3 nm) [11] , excitons are strongly confined in real space when coupling to defects [12] . Therefore, as shown theoretically for MoSe 2 and MoS 2 , chalcogen vacancy levels give rise to a series of bound defect excitons, which then hybridize with excitonic states of the pristine system [12] , [13] . At low-temperatures, most 2D semiconductors exhibit broad sub-gap emission extending several hundred meV below the exciton [4] , [5] , [7] , [8] , [14] . Generally, this sub-gap luminescence becomes stronger with increasing number of point defects present in the TMD layer, and it is often called L-band (emphasizing localization) or D-band (emphasizing defects) in the literature. The correlation between defects and the L-band was found either by introducing additional defects [5] , [14] , or by correlating spatial fluctuations of the existing defect density and excitonic properties [4] , [15] , [16] . Nevertheless, there is a surprising lack of consensus about the origin for such broad defect emission as well as about the detailed impact of specific defects on the excitonic properties. For example, some studies report a brightening of the room temperature exciton emission with increased defect density [6] , [17] , while other studies report an anticorrelation between defect density and PL yield [16] , [18] . For the low-temperature L-band, some studies emphasized radiative recombination at intrinsic point defects as underlying mechanism [4] , [7] . Other studies highlighted the relevance of molecular adsorbates. For example, calculations suggest that adsorbed molecular oxygen modifies the electronic structure of the sulfur vacancy in MoS 2 , either by removing the in-gap state [19] or by p -doping via hole transfer from the absorbed molecular oxygen [6] . In this context, a brightening of room temperature excitonic emission in MoS 2 upon oxygen plasma annealing was attributed to p-type counter-doping caused by chemisorption of oxygen radicals at sulfur defect sites, but no systematic correlation to defect emission was established [6] . Furthermore, it has been suggested that laser illumination incorporates atomic oxygen into pre-existing chalcogen vacancies either by photo-assisted dissociation of molecular oxygen [20] or water [21] . However, chalcogen vacancies are likely already passivated by atomic oxygen in as-prepared TMDs [9] , [22] , [23] . Moreover, several studies demonstrated that laser annealing in controlled gas environments [24] , [25] or encapsulation in hBN [26] can completely remove the L-band suggesting chemisorbed or physisorbed molecules as its origin [25] . By contrast, a spectrally sharp sub-gap luminescence and single photon emission was also reported at low-temperatures [2] . As the microscopic model, a combination of strain potentials, which funnel and localize excitons, and atomic defects, which provide recombination centers for localized excitons, was suggested [2] . While these point-like emitters appear randomly in as-prepared samples, they can be generated deterministically via engineered nanoscale strain potentials [2] . Recently, our group has demonstrated that atomic point defects, which are created deterministically by focused He-ion irradiation using a helium ion microscope (HIM) [9] , act as narrow and reproducible single-photon emitters, yet without a local strain potential [3] , [27] . Here, we disentangle broad defect emission due to adsorbates, which can be desorbed by in-vacuo annealing at moderate temperatures, and narrow defect emission via sulfur vacancies, which are generated both by annealing at high temperatures and He-ion irradiation. Combing controlled defect engineering with optical spectroscopy as well as atomic imaging and ab initio theory, we identify the optical signature of chalcogen vacancies in MoS 2 . 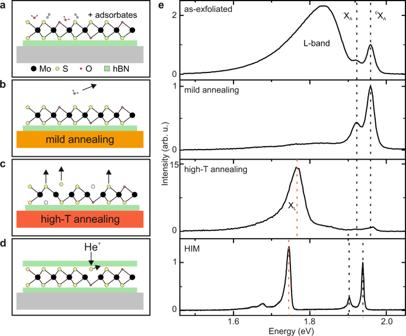Fig. 1: Optical emission induced by adsorbates and engineered point defects in single-layer MoS2. aSchematic of as-exfoliated single layer MoS2on hBN (green) supported on a Si/SiO2substrate (gray). Black (yellow) dots denote molybdenum (sulfur) atoms. Red dots denote oxygen atoms, which are present either as part of adsorbates or as substitutional atoms on sulfur sites.bHeating the substrate to mild annealing temperatures (Tannealing< 500 K, orange) removes the absorbates.cHeating the substrates to high annealing temperatures (Tannealing> 500 K, red) creates sulfur vacancies by thermal desorption (arrows).dSchematic of vacancy generation in MoS2fully encapsulated in hBN through He-ion (He+) bombardment.eEvolution of low-temperature (T∼20 K) photoluminescence spectra. As-exfoliated MoS2exhibits a broad sub-gap luminescence (L-band) due to adsorbates. Mild annealing atTannealing=  500 K removes these adsorbates suppressing the L-band. Upon annealing at Tannealing=  800 K, a narrow defect luminescence at 1.75 eV emerges (XL), due to the thermal generation of sulfur vacancies with well-defined in-gap states. Vertical, dashed lines indicate the emission energy of the neutral exciton (0XA), the trion (−XA), and XL. The intensities are normalized to the exciton transition0XA. Helium-ion (He+) irradiation of MoS2encapsulated in hBN using a helium ion microscope (HIM) generates a similar defect feature at 1.75 eV (T= 4.2 K). Defect luminescence in MoS 2 Figure 1a–d show schematic atomistic representations of MoS 2 at different stages of the annealing process. The corresponding low-temperature photoluminescence (PL) spectra of monolayer MoS 2 on hexagonal boron nitride (hBN) are depicted in Fig. 1e . In addition to exciton ( 0 X A ) and trion ( − X A ) [11] , as-exfoliated MoS 2 exhibits a prominent L-band from approximately 1.5–1.9 eV. Mild annealing ( T annealing = 500 K) in vacuum results in a striking reduction of the L-band, presumably due to desorption of adsorbates. Further annealing at high temperature ( T annealing = 800 K) introduces a narrow peak X L at approximately 1.75 eV. A similar, yet even sharper, spectral signature is observed in fully encapsulated MoS 2 after He-ion irradiation. We note that the data on the ion treated sample was measured on fully encapsulated MoS 2 with top and bottom hBN, which is necessary for the ex-situ He-ion bombardment, whereas the data on the thermally annealed sample was measured on half-encapsulated MoS 2 , with bottom hBN only. The small exciton red-shift in the He-ion treated sample can likely be attributed to the increased dielectric screening in the fully encapsulated samples [28] . Additionally, inhomogeneous broadening effects due to a locally varying dielectric environment near the defects may result in an uncertainty of the defect emission line on the order of several meV [29] , [30] . The improved inhomogeneous broadening agrees with previous studies of fully hBN encapsulated heterostructures [26] . In the following, we show that adsorbates introduce a continuum of defect states, which is responsible for the L-band emission, whereas pristine sulfur vacancies, i.e., sulfur vacancies not passivated by atomic oxygen or decorated by molecular species, introduce a deep center, which is very likely also the origin of recently discovered single photon emission in He-ion treated MoS 2 [3] , [27] . Fig. 1: Optical emission induced by adsorbates and engineered point defects in single-layer MoS 2 . a Schematic of as-exfoliated single layer MoS 2 on hBN (green) supported on a Si/SiO 2 substrate (gray). Black (yellow) dots denote molybdenum (sulfur) atoms. Red dots denote oxygen atoms, which are present either as part of adsorbates or as substitutional atoms on sulfur sites. b Heating the substrate to mild annealing temperatures ( T annealing < 500 K, orange) removes the absorbates. c Heating the substrates to high annealing temperatures ( T annealing > 500 K, red) creates sulfur vacancies by thermal desorption (arrows). d Schematic of vacancy generation in MoS 2 fully encapsulated in hBN through He-ion (He + ) bombardment. e Evolution of low-temperature ( T ∼ 20 K) photoluminescence spectra. As-exfoliated MoS 2 exhibits a broad sub-gap luminescence (L-band) due to adsorbates. Mild annealing at T annealing =  500 K removes these adsorbates suppressing the L-band. Upon annealing at T annealing =  800 K, a narrow defect luminescence at 1.75 eV emerges (X L ), due to the thermal generation of sulfur vacancies with well-defined in-gap states. Vertical, dashed lines indicate the emission energy of the neutral exciton ( 0 X A ), the trion ( − X A ), and X L . The intensities are normalized to the exciton transition 0 X A . Helium-ion (He + ) irradiation of MoS 2 encapsulated in hBN using a helium ion microscope (HIM) generates a similar defect feature at 1.75 eV ( T = 4.2 K). 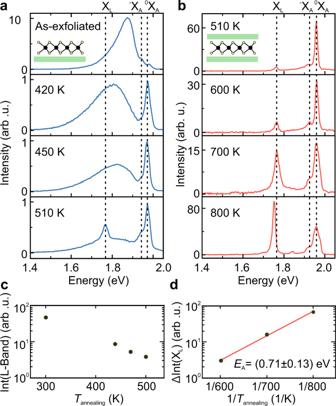Fig. 2: Evolution of MoS2low-temperature PL with increasing annealing temperature. aCompared to as-exfoliated MoS2on hBN (top panel) the broad L-band is strongly reduced after successive mild annealing. At 510 K, an emission line XLappears at 1.75 eV (bottom panel). The spectra were normalized to the intensity of the exciton to highlight relative changes between the L-band, the trion and the free exciton emission.bPL spectra of fully encapsulated MoS2. With increasing annealing temperature, the intensity of XLincreases. Dashed lines highlight neutral exciton (0XA), trion (−XA), and XL. The spectra are presented as measured without further normalization.cIntegrated intensity of the L-band inaas function of annealing temperature. The change in L-band emission is related to the desorption rate of adsorbates from the MoS2.dArrhenius plot of thermal defect generation rate extracted from the change in intensity of XLbetween subsequent annealing steps, which is denoted as ΔInt(XL). The activation barrierEAextracted from the fit (red line) is (0.71 ± 0.13) eV consistent with formation of sulfur vacancies. Full size image Defect luminescence induced by thermal annealing Figure 2 shows low-temperature PL of MoS 2 after stepwise in-vacuo annealing up to 800 K. In each cycle, the samples were rapidly annealed in a customized cryostat for 30 min, and then cooled back to cryogenic temperature ( T sample ∼ 20 K) for PL characterization maintaining a high vacuum ( p < 10 −4 mbar) at all times (Supplementary Note 1 ). Figure 2a illustrates spectra of as-exfoliated MoS 2 on hBN and after several mild annealing steps to 420, 450, and 510 K. Again, the as-exfoliated flake exhibits a prominent L-band (cf. Fig. 1a ). The intensity of the L-band decreases relative to the intensity of the free exciton emission by one order of magnitude after annealing to T annealing = 420 K, and it gradually disappears for higher annealing temperatures (Fig. 2b ). Furthermore, the trion emission decreases initially compared to the free exciton indicating a reduced doping, as observed previously in TMDs during desorption of physisorbed gas [31] and chemical dopants [32] . Hence, we attribute the L-band to adsorbates, which are progressively removed during the mild annealing steps. The desorption does not follow a simple Arrhenius law, since it depends on the total number of adsorbates, which is unknown. Therefore, we can estimate only an upper bound of ~100 meV for the desorption barrier, which agrees with ab initio studies for molecular adsorbates on MoS 2 [33] and temperature programmed desorption on bulk MoS 2 [34] . Fig. 2: Evolution of MoS 2 low-temperature PL with increasing annealing temperature. a Compared to as-exfoliated MoS 2 on hBN (top panel) the broad L-band is strongly reduced after successive mild annealing. At 510 K, an emission line X L appears at 1.75 eV (bottom panel). The spectra were normalized to the intensity of the exciton to highlight relative changes between the L-band, the trion and the free exciton emission. b PL spectra of fully encapsulated MoS 2 . With increasing annealing temperature, the intensity of X L increases. Dashed lines highlight neutral exciton ( 0 X A ), trion ( − X A ), and X L . The spectra are presented as measured without further normalization. c Integrated intensity of the L-band in a as function of annealing temperature. The change in L-band emission is related to the desorption rate of adsorbates from the MoS 2 . d Arrhenius plot of thermal defect generation rate extracted from the change in intensity of X L between subsequent annealing steps, which is denoted as ΔInt(X L ). The activation barrier E A extracted from the fit (red line) is (0.71 ± 0.13) eV consistent with formation of sulfur vacancies. Full size image At T annealing = 510 K, a spectrally narrow emission line X L appears around 1.75 eV. In contrast to the L-band, the intensity of X L increases with higher annealing temperatures, until the whole PL signal disappears at T annealing > 700 K (Supplementary Note 2 ). To extract the thermal activation barrier of X L , we use an hBN/MoS 2 /hBN heterostack, where the L-band is already suppressed in the as-prepared structures. As seen in Fig. 2c , X L brightens in the encapsulated monolayer with increasing annealing temperature, and further narrows after annealing to 800 K indicating a complete removal of residual adsorbates. At even higher temperatures ( T annealing = 900 K), the intensity of X L decreases drastically, followed by the complete disappearance of the overall PL (Supplementary Note 2 ). Consistent with saturating a finite density of localized defect levels, X L exhibits a saturating behavior as function of excitation power (Supplementary Note 3 ) [27] . In a simple rate equation model, the saturated defect emission is then proportional to the total number of emission centers. In this case, we can readily determine the energy barriers for defect generation since it is proportional to the difference in the integrated spectral weight of X L compared to the previous annealing step. For example, the number of defects generated during annealing at 600 K is proportional to the difference in integrated PL intensity, which we label ΔInt(X L ), after annealing to 600 and 510 K. In the limit of low density, defect generation is independent of the number of existing defects, and we expect a simple Arrhenius law. From Fig. 2d , we find an activation energy of (0.71 ± 0.13) eV for the X L -peak consistent with theoretical predictions for the formation energy of mono-sulfur vacancies (approximately 1 eV) [35] , [36] . The error was calculated from the standard deviation of the fit parameter for the slope. Interstitial sulfur defects should not form under high-vacuum, i.e., sulfur-poor, conditions [35] . The formation energies for transition metal vacancies are much larger (3–8 eV) [35] , [36] . Consequently, the formation of sulfur vacancies during annealing is thermodynamically the most favorable and, therefore, most likely process. To independently corroborate the value of the thermal activation energy and to quantify the absolute number of defects generated at a given temperature, we conducted a Raman study of additional, thermally annealed samples (Supplementary Note 4 ). At large enough defect densities, the inter-defect distance, or equivalently the absolute value of the defect density, can be inferred from a shift of the characteristic Raman modes due to phonon confinement effects [30] , [37] , [38] . From these experiments we extract an activation energy of (0.48 ± 0.23) eV for thermal defect generation, which agrees well with our in-situ study within the experimental uncertainty. For high annealing temperatures ( T annealing = 900 K), we can even determine the absolute value of the reaction rate to be on the order of 5 × 10 13 vacancies per cm² per hour. However, we note that this value should only serve as a rough order of magnitude estimate. Atomic-scale identification of sulfur vacancy defects We continue to corroborate the dominant generation of sulfur vacancies during annealing by atomic-scale characterization. Here, we perform high-resolution low-temperature scanning tunneling microscopy (STM) and atomic force microscopy (AFM) of single-layer MoS 2 before and after high-temperature annealing in vacuum ( T annealing > 500 K) as well as before and after He-ion irradiation. These experiments are conducted on graphene/SiC heterostructures. The graphene substrate is essential as conductive support, but it quenches the defect emission, which is slow (100 ns–1 µs) [3] , [29] , [30] , and therefore the fast exciton emission (~10 ps) dominates on graphene (Supplementary Note 5 ) [16] , [39] . For STM, all samples were prepared in-vacuo by a mild annealing step in vacuum ( T annealing < 500 K) to remove adsorbates. Several STM studies established correlations between defect densities and (opto)electronic material properties of transition metal dichalcogenides, via large scale imaging at moderate resolution and counting of localized features [18] , [40] , [41] . In the following, we focus on the exact identification of atomic defects via high-resolution imaging of the orbital structure as well as independent corroboration of the lattice site, via AFM and ab initio simulations [22] . In agreement with our optical studies, the surface of MoS 2 is virtually free from adsorbates after mild annealing. By far the most dominant defects in pristine material were oxygen atoms substituting sulfur, but no sulfur vacancies were observed within our statistics (Supplementary Note 6 ) [9] , [22] , [23] . The latter observation is in line with previous studies on MoSe 2 grown by molecular beam epitaxy and WS 2 grown by chemical vapor deposition, where in as-grown samples the dangling bonds of sulfur vacancies are effectively passivated by chemically bound atomic oxygen in the trigonal lattice configuration of the transition metal dichalcogenide [22] , [23] . After additional high-temperature annealing, we observed only two additional types of defects within our experimental statistics (Fig. 3 ). Their high-resolution STM topography exhibits a trigonal symmetry (Fig. 3a, b ), consistent with a vacancy either in the top or bottom sulfur lattice. For both vacancies, the charge densities calculated by DFT (Supplementary Note 7 ) at a distance of 4.5 Å above the MoS 2 layer (similar to experimental conditions in STM) are shown in Fig. 3c, d . The calculations are in good agreement with the STM topography. The top vacancy appears trigonally ring-shaped, whereas the bottom vacancy appears triangular-shaped with bright maxima at the corners. These same defects, i.e., top and bottom sulfur vacancies, were also confirmed in the He-ion irradiated samples (Fig. 3e, f ). 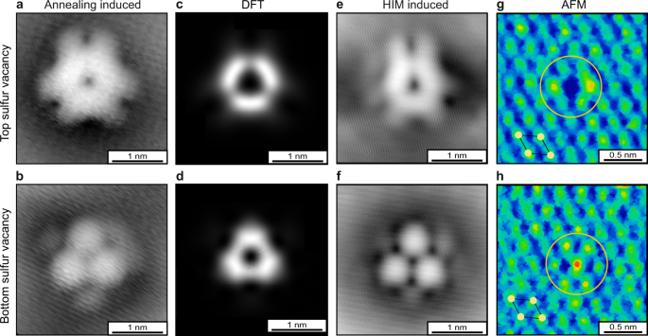Fig. 3: Scanning probe microscopy of sulfur vacancies in single-layer MoS2on graphene. a,bScanning tunneling microscope (STM) images of annealing induced vacancies in the top and bottom sulfur layer. The STM imaging parameters were tip biasVbias= 450 mV, tunneling currentIt= 100 pA.c,dDensity functional theory (DFT) calculations of 7 × 7 supercell containing one sulfur vacancy. The image displays a constant height slice 4.5 Å above and below the MoS2layer corresponding to the charge density from sulfur vacancies in the top and bottom sulfur layer, respectively.e,fSTM images of He-ion (HIM) induced top and bottom sulfur vacancies.g,hAtomic force microscopy (AFM) images of the top and bottom sulfur vacancies. The centers of the circles highlight the position of the vacancy defect. The pictogram indicates the sulfur lattice (yellow dots). For He-ion treated samples, sulfur vacancies are the dominant defect type, among other defects that are generated with lower yield [9] . Furthermore, we performed CO-tip AFM on the sulfur vacancies (Fig. 3g, h ). For the top vacancy, we observe an apparent depression at the sulfur site, whereas for the bottom vacancy structural relaxation results in a slight protrusion, in agreement with previous studies on WS 2 [23] . Most importantly, AFM conclusively assigns the defect onto the sulfur sublattice, which is difficult from STM alone [20] . Overall, the scanning probe experiments confirm the composition and surface condition of MoS 2 derived from optical characterization (cf. Fig. 1 ). From our different annealing experiments, we conclude that defect luminescence X L at 1.75 eV arises from pristine, i.e., undecorated, sulfur vacancies. We note that, there are at least two pathways for formation of sulfur vacancies, which are desorption of a sulfur atom or desorption of an oxygen atom from a sulfur site. The latter substitute for sulfur in as-prepared TMDs [22] , [23] . Based on the similarity of the optical spectra and the abundance of sulfur vacancies in thermally annealed as well as in He-ion irradiated MoS 2 (cf. Fig. 1 ), we propose that also the origin of quantum emission from individual He-ion induced defects is due to the (non-passivated) sulfur vacancy [27] . Fig. 3: Scanning probe microscopy of sulfur vacancies in single-layer MoS 2 on graphene. a , b Scanning tunneling microscope (STM) images of annealing induced vacancies in the top and bottom sulfur layer. The STM imaging parameters were tip bias V bias = 450 mV, tunneling current I t = 100 pA. c , d Density functional theory (DFT) calculations of 7 × 7 supercell containing one sulfur vacancy. The image displays a constant height slice 4.5 Å above and below the MoS 2 layer corresponding to the charge density from sulfur vacancies in the top and bottom sulfur layer, respectively. e , f STM images of He-ion (HIM) induced top and bottom sulfur vacancies. g , h Atomic force microscopy (AFM) images of the top and bottom sulfur vacancies. The centers of the circles highlight the position of the vacancy defect. The pictogram indicates the sulfur lattice (yellow dots). Full size image Excitonic defect states from ab initio theory In a simple single-particle picture, three types of excitonic transitions can be qualitatively distinguished (Fig. 4a ), similar to the approaches in ref. [12] for MoSe 2 and ref. [42] for WSe 2 . However, taking many-body effects into account, the strong electron–hole interaction leads to a vast manifold of excitonic transitions for the defective crystal with varying eigenenergies and mixed degrees of pristine and defect-like character, which all contribute to the excitonic spectrum [12] , [13] . 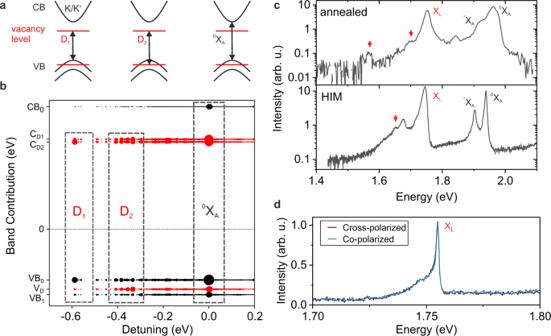Fig. 4: Defect bound excitons in monolayer MoS2. aQuasiparticle conduction (CB) and valence (VB) bands (black) near K-points and K′-points in the Brillouin zone of single-layer MoS2. The red lines denote states arising from sulfur vacancy levels. Arrows highlight the three types of excitonic transitions: between the delocalized bands (0XA), between the localized defect states only (D2) and between the valence band and the localized defect state (D1).bBand contribution to exciton transitions computed with GW-BSE. Dot size represents the relative oscillator strength, and the probability amplitudes of the occupied and empty bands contributing to it. Black indicates delocalized band states and red indicates localized defect states. CB0and VB0, VB1denote the dispersive unoccupied conduction and occupied valence bands (above and below the Fermi level), respectively. CD1and CD2are unoccupied localized defect levels, split by spin–orbit interaction arising from conduction band states.VDis the occupied localized defect level arising from the valence band. The three main peaks regions assigned with the D1,D2, and0XAtransitions are marked with dashed lines.cPL spectra of annealed and HIM-treated MoS2. The defect emissions occur in a range of 0.2–0.3 eV below XAwith a dominant emission line (XL) around 1.75 eV. Further features (red arrows) are resolved at even larger detuning from the free exciton, in qualitative agreement with the predicted continuum of excitonic defect states below the pristine optical gap.dA single He-ion induced emitter shows no detectable valley polarization (T=  10 K, excitation energy 2.1 eV) as expected for transitions involving only defect levels (D2). Figure 4b shows the excitonic spectrum and its band contributions from calculations of defective MoS 2 (5 × 5 supercell corresponding to 2% of vacancies) within the GW-Bethe–Salpeter equation (GW-BSE) approach [43] , [44] . Each set of dots at a given energy describes an excitonic eigenstate of the defective MoS 2 crystal. The size of the dots is proportional to the contributions from different bands, integrated across the Brillouin zone, to a particular excitonic state. This detailed evaluation of the band contributions suggests that transitions at the optical gap ( 0 X A ) have a substantial component from unbound electronic states between valence and conduction bands at K and K′ valleys (see also Supplementary Note 8 ). The next series of transitions (D 2 ) occur predominantly between the resonant defect state overlapping with the valence band and the localized in-gap states. In the dilute limit, the localized defect states are k-independent, such that defect–defect transitions cannot exhibit valley-selectivity [12] . The lowest series of transitions (D 1 ) couples the localized in-gap state to dispersive states in the valence band near K and K′, and they are predicted to show valley selectivity and corresponding polarization. Fig. 4: Defect bound excitons in monolayer MoS 2 . a Quasiparticle conduction (CB) and valence (VB) bands (black) near K-points and K′-points in the Brillouin zone of single-layer MoS 2 . The red lines denote states arising from sulfur vacancy levels. Arrows highlight the three types of excitonic transitions: between the delocalized bands ( 0 X A ), between the localized defect states only (D 2 ) and between the valence band and the localized defect state (D 1 ). b Band contribution to exciton transitions computed with GW-BSE. Dot size represents the relative oscillator strength, and the probability amplitudes of the occupied and empty bands contributing to it. Black indicates delocalized band states and red indicates localized defect states. CB 0 and VB 0 , VB 1 denote the dispersive unoccupied conduction and occupied valence bands (above and below the Fermi level), respectively. C D1 and C D2 are unoccupied localized defect levels, split by spin–orbit interaction arising from conduction band states. V D is the occupied localized defect level arising from the valence band. The three main peaks regions assigned with the D 1, D 2 , and 0 X A transitions are marked with dashed lines. c PL spectra of annealed and HIM-treated MoS 2 . The defect emissions occur in a range of 0.2–0.3 eV below X A with a dominant emission line (X L ) around 1.75 eV. Further features (red arrows) are resolved at even larger detuning from the free exciton, in qualitative agreement with the predicted continuum of excitonic defect states below the pristine optical gap. d A single He-ion induced emitter shows no detectable valley polarization ( T =  10 K, excitation energy 2.1 eV) as expected for transitions involving only defect levels (D 2 ). Full size image In Fig. 4c , we show experimental PL emission spectra of MoS 2 with vacancies, introduced in encapsulated MoS 2 both by in-vacuo thermal annealing and by ex-situ helium ion modification. Notably, while the dominant defect emission (X L ) occurs about 0.2 eV below 0 X A , we consistently observe weak emission features (red arrows) at even lower energies [3] . The multiple sub-gap emission peaks are qualitatively in agreement with the manifold of exciton states predicted by the calculations of the defective MoS 2 (Fig. 4b ). The calculated absolute energy of the features associated with transitions of type D 2 is centered at 1.8 eV, which is consistent with defect emission at 1.75 eV, within the overall computational uncertainty on the order of 0.2 eV (Supplementary Note 9 ). Figure 4c further corroborates this assignment. Here, we plot the emission spectrum of a single defect, which was generated by He-ion bombardment [9] , [27] , for co-circularly and cross-circularly polarized excitation and detection. We do not detect a valley polarization, as expected for a transition that occurs predominantly between localized defect levels. We note that the absence of valley polarization for defect emission in monolayer transition metal dichalcogenides is non-trivial. For example, Hsu et al. reported a valley polarization for defect localized excitons in CVD-grown WSe 2 [45] . Similarly, Moody et al. reported valley polarization of defect localized excitons in exfoliated, electron beam irradiated WSe 2 [42] , which they assigned to defect-to-valence-band transitions. In both works, the defect emission was rather broad (about 60–100 meV) and the samples were neither in-situ prepared or encapsulated, such that adsorbates may have contributed to the observed defect emission. For clean and low-defect density WSe 2 , excitonic satellite peaks were recently demonstrated and assigned to bound-excitons complexes localized by residual unintentional dopants. In the latter study, a valley polarization of the satellite peak was observed as well [46] . In our case, we conclude that the X L peak observed in our thermally annealed as well as He-ion treated MoS 2 monolayers arises, due to a localized excitonic transition between the defect orbitals of the pristine sulfur vacancy. Typically, the dominant emission process should involve the lowest energy state of the system, i.e., transitions of type D 1 , which according to the theoretical results may allow accessing defect-related valley polarizations in the Brillouin zone via their valley contributions near K and K′ (see also Supplementary Note 8 ). However, in our experiments, the defect emission is governed by transitions of intermediate energy, i.e., transitions of type D 2 , although the calculated oscillator strength varies only weakly in the relevant regime. A naïve scenario to explain our observations involves a relaxation cascade after the absorption process: optical excitation creates a free exciton, which gets localized, and then both hole and electron decay into a defect state (type D 2 ). If further relaxation of the captured exciton into an excitonic state of type D 1 is slow or prohibited, the emission will occur dominantly from the fully localized electron and hole state. From a theory point of view, the above picture demands not only going from absorption to emission, but also to include further interactions, such as exciton–exciton or exciton–phonon coupling [47] . The latter is motivated by the fact that previous work described the asymmetric line shape of defect emission by an independent boson model with a phonon bath [27] . Furthermore, in a recent study [30] , we found signatures of phonon replica corresponding to Raman shift of 248 cm −1 suggesting that the defect emission can couple also to localized optical phonon modes. Overall, these insights can provide starting points for the theoretical description of emission properties of such atomistic defects in highly confined two-dimensional material systems. In summary, by combining far-field optical spectroscopy, atomic-resolution scanning probe microscopy, and ab initio theory, our study provides compelling evidence of optical defect emission from pristine sulfur vacancies in single layer MoS 2 . In contrast to previous studies, these pristine sulfur vacancies are generated in-vacuo or capped by hBN, and therefore, neither passivated by oxygen nor decorated with adsorbates. Similar to previous reports, we observe a broad L-band luminescence due to adsorbates in as-prepared MoS 2 monolayers, which can be suppressed by a combination of h-BN encapsulation and mild annealing. In as-prepared layers and after mild annealing, pristine sulfur vacancies are absent, and oxygen passivated vacancies are the dominant defect. We suggest that oxygen-passivated vacancies form active sites for adsorption of molecular species, since many previous studies established a positive correlation between sulfur deficiency and defect emission [4] , [5] , [15] . Pristine vacancies are created in h-BN/MoS 2 /h-BN heterostructures either via in-vacuo thermal annealing or ex-situ helium ion bombardment, whereby the latter allows generating single photon emitters on demand [27] with a position accuracy below 10 nm [9] . Guided by ab initio calculations, we identify transitions between a localized in-gap defect state and a localized resonant defect state as the most likely candidate. Sample preparation We micromechanically exfoliated synthetic MoS 2 and hBN (NIMS, K.W. and T.T.) using adhesive tape. We used an all-dry viscoelastic stamping technique to transfer single flakes to a substrate consisting of SiO 2 /Si for PL characterization or epitaxial graphene on (6H)-SiC for STM/AFM characterization using a polydimethylsiloxane (PDMS) stamp. During the transfer, we heated the samples to approximately 60 °C, to increase the transfer probability. We cleaned the samples with acetone, isopropanol, and nitrogen gas after each stacking step to remove residues and increase the adhesion. In-vacuo annealing For PL characterization, we annealed the MoS 2 /hBN/SiO 2 samples in a modified optical cryostat (Janis ST-500). A customized heater was added to the cryostat for rapid thermal cycling between cryogenic temperatures ( T sample ∼ 20 K) and high temperatures ( T sample ∼ 900 K). We determined the annealing temperature at the sample with a thermocouple. We rapidly ramped to the desired annealing temperature and kept it constant for 30 min, then we cooled the sample with the highest possible rate back to cryogenic temperatures and conducted the PL measurements. Photoluminescence spectroscopy The annealed samples (Figs. 1a–c , 2 , and 4c ) were studied with a custom microscope set-up ( λ excitation = 532 nm, Nikon Plan Fluor ELWD 20×/0.45, WD 7.4 mm). The cryostat was mounted on a motorized xy-stage (ASI) with a minimum stepsize of 100 nm. The emitted light was focused onto the entrance slit of the spectrometer (Andor Kymera 328, grating 300 grooves/mm), and the signal was collected by a CCD camera (Andor iXon). The photoluminescence of the ion-treated samples (Figs. 1d and 4c , d ) was measured in a He-flow cryostat at T = 4.2–10 K ( λ excitation = 590 nm, Mitutoyo 100x/0.5 M Plan Apo NIR, WD 12 mm, PI Acton SP-2500i spectrometer, grating 300 grooves/mm). For valley polarization measurements, the circular polarization was adjusted using an achromatic λ/4-plate in front of the objective lens. The emitted light passed again through the same waveplate, and the polarization was analyzed using a linear polarizer. Scanning probe microscopy We performed combined scanning tunneling microscopy and atomic force microscopy (Createc) at low temperatures ( T ∼ 6 K) in vacuum with a base pressure of around 10 −10 mbar. For STM/AFM, the MoS 2 /graphene/SiC samples were treated by mild annealing ( T ∼ 500 K) under UHV conditions for 10–20 min. All STM images were recorded using the constant-current feedback and current setpoint of I t = 100 pA. Chemically etched tungsten tips were sharpened by repeated indentations into a Au(111) substrate. All AFM images were recorded with a qPlus quartz crystal tuning fork in constant height mode with an applied bias voltage V bias = 0 V. Helium ion microscopy Single layer MoS 2 flakes supported by graphene/SiC were nanostructured using a helium ion microscope (HIM ORION NanoFab, Zeiss). The whole MoS 2 flake was exposed to a constant helium ion dose of 5 × 10 14 cm −2 . We operated the HIM at a helium pressure of 2.5 × 10 −6 Torr, a beam energy of 30 keV, beam current of 0.7 pA, pixel spacing of 5 nm, and field of view (FOV) of 100 µm. To obtain the desired constant helium ion dose, the dwell time was adapted to the beam current. Ex-situ annealing and Raman spectroscopy For ex-situ annealing studies, samples were annealed in a rapid thermal annealer under nitrogen atmosphere at a pressure of several mbar for 30–60 min at varying temperatures from 400 to 950 K. The cooling and heating ramp rate were about 10 K/s. After the annealing, the samples were taken out, exposed to ambient, and transferred into a vacuum chamber (base pressure < 10 −5 mbar) for optical characterization. For Raman spectroscopy at room temperature, we used a WiTec Alpha 300 microscope (Zeiss Neofluar 60×, 0.6 NA with correction collar, 532 nm excitation wavelength, P laser = 0.3 mW). Theoretical calculations DFT calculations of the defect orbitals in Fig. 3 were performed using the Vienna Ab initio Simulation Package, VASP 5.4.4 [48] . Details can be found in Supplementary Note 7 . The GW-BSE calculations of the excitonic spectra of MoS 2 with sulfur vacancies, shown in Fig. 4 , were performed using the Quantum Espresso [49] and the BerkeleyGW [50] packages. The computational details are described in Supplementary Note 9 .